Highly deformable liquid-state heterojunction sensors Mechanically deformable devices and sensors enable conformal coverage of electronic systems on curved and soft surfaces. Sensors utilizing liquids confined in soft templates as the sensing component present the ideal platform for such applications, as liquids are inherently more deformable than solids. However, to date, liquid-based devices have been limited to metal lines based on a single-liquid component given the difficulty in the fabrication of liquid-based junctions due to intermixing. Here, we demonstrate a robust platform for the fabrication of liquid–liquid ‘heterojunction’ devices, presenting an important advancement towards the realization of liquid-state electronic systems. The device architecture and fabrication scheme we present are generic for different sensing liquids, enabling demonstration of sensors responsive to different stimuli. As a proof of concept, we demonstrate temperature, humidity and oxygen sensors by using different ionic liquids, exhibiting high sensitivity with excellent mechanical deformability arising from the inherent property of the liquid phase. Electronic devices and sensors that exhibit large amounts of mechanical deformability have many applications in smart wallpapers [1] , [2] , physiological body sensors [3] , [4] , [5] , [6] , [7] , and human-machine interfaces for prosthetics [8] , [9] , [10] and robotics [11] , [12] , [13] , [14] . In this regard, tremendous advancements have been made in engineering solid-state electronic materials and devices on elastic substrates [1] , [6] , [9] , [10] , [15] , [16] , [17] , [18] , [19] , [20] , [21] , [22] . Recently, sensors based on using liquid active components embedded within soft elastomeric substrates have shown much promise for such applications as liquids present the ultimate limit in deformability. Previous works have shown that InGa eutectic metal can be patterned as conductive electrodes [14] , [18] , [19] , [20] , [21] , [22] and configured as pressure sensors [14] , capable of withstanding up to 250% strain without failure. One limiting factor in the fabrication of more sophisticated liquid-based sensors is the inability to combine multiple liquids into one device due to intermixing. Through modelling and experiments, we present the design requirements for the device architecture and the liquid properties needed to overcome this barrier and enable heterojunction confinement without intermixing. As a proof of concept and to show the generic nature of our design, we utilize multiple different ionic liquids as the active sensing liquid to sense different stimuli including temperature, humidity and oxygen gas sensing, with excellent performance characteristics even when under deformation. Selection of liquids Galinstan is a eutectic metal that is composed of 68.5% Ga, 21.5% In and 10% Sn. It exhibits high electrical conductivity (3.40 × 10 6 S m −1 ; ref. 21 ), low vapour pressure (<100 pPa at 25 °C; ref. 23 ) and is non-toxic [22] . These physical properties present Galinstan as an ideal liquid metal for liquid-state device applications. While Galinstan makes for an excellent conductor, it alone is not sufficient to achieve sophisticated liquid-based electronic devices. For the realization of liquid-state devices, and eventually systems, controlled heterojunctions must be made between different liquid components [24] , analogous to metal/semiconductor or semiconductor/semiconductor junctions seen in traditional solid-state devices. More generally, junctions represent the fundamental building blocks for any device technology. With this in mind, we present a fabrication platform for the controlled formation of liquid–liquid ‘heterojunctions’ using immiscible liquids. As example systems, we demonstrate the functionality of liquid heterojunctions for temperature, humidity and oxygen gas sensing. Here, Galinstan is used as the source/drain metal electrodes to contact an ionic liquid that serves as the active sensing element. Four different ionic liquids were used to enable the desired sensing functionalities, including 1-ethyl-3-methylimidazolium trifluoromethanesulfonate ([EMIM][Otf]), 1-hexyl-3-methylimidazolium chloride ([HMIM][Cl]), 1-butyl-3-methylimidazolium hexafluorophosphate ([BMIM][PF6]) and 1-butyl-1-methylpyrrolidinium bis(trifluoromethylsulfonyl)imide ([BMPYR][NTf2]). The first two ionic liquids are hydrophilic and the latter two are hydrophobic. While the resistivity of Galinstan has minimal dependence on the various stimuli explored in this work, the conductance and capacitance of the ionic liquids are highly responsive to the desired stimuli, thus providing a reliable sensor technology that can undergo severe forms of mechanical deformation without degradation or irreversible change in electrical properties. In this liquid–liquid ‘heterojunction’ concept, it is critical to prevent intermixing of the two liquid components, especially during fabrication as well as when the completed devices undergo mechanical deformation. To prevent breakdown of liquid heterointerfaces, two important design considerations are made. First, the two liquids are selected such that they are immiscible. Second, the layout and dimensions of the polydimethylsiloxane (PDMS) microfluidic template, which dictate the device architecture, are properly engineered. For the metal electrodes, we chose Galinstan owing to the reasons stated previously. For the active sensing elements, ionic liquids were chosen since they are immiscible with Galinstan. Furthermore, ionic liquids generally have a high boiling point [25] , low vapour pressure [26] and are non-flammable [27] . A high boiling point and low vapour pressure are critical to the stability of the device while operating at elevated temperatures. Given the extremely small volume of liquid (~315 nl) contained in the active region of the device, high vapour pressure liquids such as water readily evaporate through the PDMS substrate. Since ionic liquids have a nearly negligible vapour pressure, they are non-volatile without any noticeable loss through the PDMS microfluidic template for temperatures up to 80 °C. Device architecture and fabrication scheme The device was fabricated via traditional microfluidic process technology ( Fig. 1a–n ). The PDMS channels were patterned and cured on an SU-8 master mould. The patterned PDMS was then bonded onto a second unpatterned PDMS substrate to complete the formation of the microchannels. After bonding, Galinstan and the ionic liquid were injected into the channels sequentially using a syringe pump. Finally, the channels were sealed off using silicone rubber. An optical image of a fully fabricated device is shown in Fig. 1o . 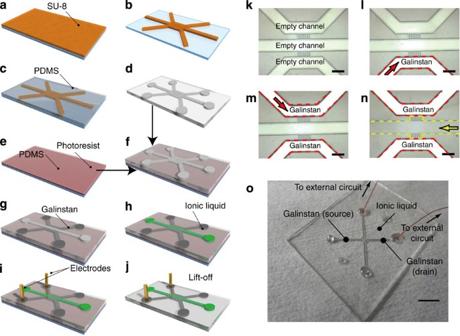Figure 1: Liquid heterojunction device fabrication. (a–j) Fabrication process flow. (k–n) Step-by-step optical microscope images taken after injection of each liquid component (scale bars, 500 μm). (o) Fully fabricated liquid heterojunction device consisting of an ionic liquid active channel and GaInSn source/drain electrodes (scale bar, 2.5 mm). Figure 1: Liquid heterojunction device fabrication. ( a – j ) Fabrication process flow. ( k – n ) Step-by-step optical microscope images taken after injection of each liquid component (scale bars, 500 μm). ( o ) Fully fabricated liquid heterojunction device consisting of an ionic liquid active channel and GaInSn source/drain electrodes (scale bar, 2.5 mm). Full size image To prevent the liquids from interpenetrating during the fabrication process or due to applied strain, we implemented high flow resistance structures at the interface of the two liquids [14] . Rather than one continuous junction connecting Galinstan and the ionic liquid, the two liquids are connected via a series of ‘heterojunction’ microchannels 30 μm wide, 31 μm high and 200 μm long ( Fig. 1k–o ). These channels, termed as junction channels, introduce regions of high flow resistance that prevent the two liquids from interpenetrating. For maximum robustness, it is ideal to design the junction channels with minimal width and height. To tune the contact area between the Galinstan and ionic liquid (that is, total junction width), the number of junction channels can be changed. Next, we explore the device design rules needed to enable fabrication of the liquid heterojunctions. The first criterion is that Galinstan must not penetrate into the junction channels (designated for ionic liquids) during injection. Two variables that affect this criteria are the total pressure P T of Galinstan and the capillary pressure P C at the junction channel interface. The total pressure is composed of the static pressure P S , which is constant for our structure, and the dynamic pressure P D , which depends on the Galinstan injection velocity, v , as described by the equation: where ρ is the density of Galinstan (6.44 g cm −3 ) and v is controlled by the volume injection rate of the syringe pump. The capillary pressure is the pressure drop across the Galinstan–air interface and is calculated using the equation: where θ is the contact angle of Galinstan on PDMS and is measured to be 134° using a Kruss contact angle analyser ( Fig. 2a ), which is in line with reported values of 120–140° in literature [28] . The phenomenological parameter γ is a measure of the force between the Galinstan and the PDMS surface, and w and h are the width and height of the junction channel, respectively. In order for Galinstan to not enter the junction channels during injection, P T must be less than P C ( Fig. 2b ). 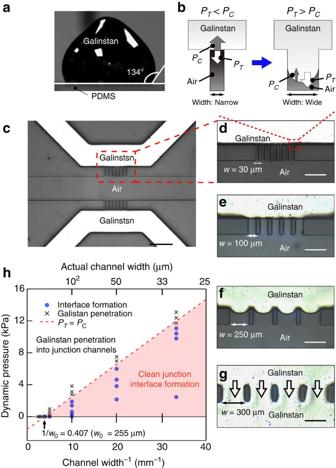Figure 2: Design considerations for the fabrication of liquid heterojunctions. (a) Contact angle of Galinstan on oxygen plasma-treated PDMS, measured to be 134°. (b) Schematic illustrations of narrow and wide junction channels during Galinstan injection, depicting the relationship between the capillary pressure (PC) and total pressure (PT). For the narrow junction channels, wherePT<PC, the heterojunction is successfully formed. However, for the wide junction channels, wherePT>PC, Galinstan penetrates into the junction channels, preventing controlled formation of the heterojunction. (c) Optical image of a device after Galinstan injection (scale bar, 500 μm). The separation of Galinstan from the junction channel edge (before the injection of ionic liquid) is maintained for devices with junction widths (d) 30, (e) 100 and (f) 250 μm. (g) In the case of a device withw=300 μm, Galinstan penetrates into the area designated for the ionic liquid. Scale bars, 250 μm (d–g). (h) The relationship between dynamic pressure and the inverse of the junction channel width. Different dynamic pressures at each channel width correspond to different injection velocities of Galinstan.W0is the structural limit extracted from thex-intercept of the linear regression of the experimental lower bounds of dynamic pressure for which Galinstan penetrates into the junction channels. Figure 2: Design considerations for the fabrication of liquid heterojunctions. ( a ) Contact angle of Galinstan on oxygen plasma-treated PDMS, measured to be 134°. ( b ) Schematic illustrations of narrow and wide junction channels during Galinstan injection, depicting the relationship between the capillary pressure ( P C ) and total pressure ( P T ). For the narrow junction channels, where P T < P C , the heterojunction is successfully formed. However, for the wide junction channels, where P T > P C , Galinstan penetrates into the junction channels, preventing controlled formation of the heterojunction. ( c ) Optical image of a device after Galinstan injection (scale bar, 500 μm). The separation of Galinstan from the junction channel edge (before the injection of ionic liquid) is maintained for devices with junction widths ( d ) 30, ( e ) 100 and ( f ) 250 μm. ( g ) In the case of a device with w =300 μm, Galinstan penetrates into the area designated for the ionic liquid. Scale bars, 250 μm ( d – g ). ( h ) The relationship between dynamic pressure and the inverse of the junction channel width. Different dynamic pressures at each channel width correspond to different injection velocities of Galinstan. W 0 is the structural limit extracted from the x -intercept of the linear regression of the experimental lower bounds of dynamic pressure for which Galinstan penetrates into the junction channels. Full size image To further shed light on the model above and experimentally obtain the quantitative parameters needed for successful device fabrication, we varied w and v to modulate P C and the dynamic pressure component of P T , respectively. Specifically, w was varied from 30 to 300 μm while the height and length were fixed at 31 and 200 μm, respectively. The injection rate for Galinstan was varied from 25 to 1,900 μl min −1 . Optical microscope images of representative devices with different w fabricated using v =27 mm s −1 are shown in Fig. 2c–g . As evident from the images, Galinstan is confined to the designed electrode regions when w <250 μm ( Fig. 2d–f ). However, the Galinstan interface does not maintain its integrity when w >250 μm ( Fig. 2g ). While it is possible to use the pressure of the ionic liquid injection to push the Galinstan back to its own territory for channels with w ~250 μm, where there is partial invasion into the junction channels, we find that doing so does not result in sharp junctions ( Supplementary Fig. 1 ). Thus, it is best to use w as the main fabrication parameter for creating well-defined junction interfaces. Figure 2h shows the relationship between dynamic pressure (obtained by varying v ) and the inverse of the junction channel width, w −1 in determining the fabrication success of the devices. The linear regression, extracted from the experimental lower bounds of dynamic pressure for Galinstan penetration into the junction channels, corresponds to the limit at which P C = P T = P D + P S . From the slope of the regression line, we extract γ =600±86 (mN m −1 ), which is comparable to previously reported values of 624–630 mN m −1 (ref. 18 ). The x -intercept of the regression indicates the structural limit of the junction channel width ( W 0 ), extracted to be 255 μm. This represents the maximum junction width for which Galinstan diffusion into the active device area can be blocked as v , and thereby P D , approaches zero. In addition to proper channel design, the order of liquid injection during the fabrication process is important. Ionic liquids have a low contact angle with PDMS ( Supplementary Fig. 2 ) which means that P C is directed in the same direction as P T . As a result, ionic liquids invade all patterned channels, including those designated for the Galinstan electrodes ( Supplementary Fig. 3 ) via capillary pressure if injected first, regardless of the junction channel dimensions or injection velocity. On the other hand, given the high contact angle of Galinstan on PDMS (~134°), it can be controllably injected into the designated regions as long as the proper design parameters for the junction channels are incorporated as previously discussed. Thus, Galinstan is injected before the ionic liquid. After Galinstan patterning, the ionic liquid is injected into the active channel region to complete the liquid heterojunction. Once again, owing to the direction of the capillary pressure, the ionic liquid naturally diffuses into the junction channels until it interfaces with Galinstan, completing the controlled formation of liquid–liquid junctions between Galinstan and the ionic liquid. While other liquid parameters such as viscosity may have a slight role, their effects are minimal ( Supplementary Fig. 2 ). Liquid-state devices exhibit excellent mechanical deformability. 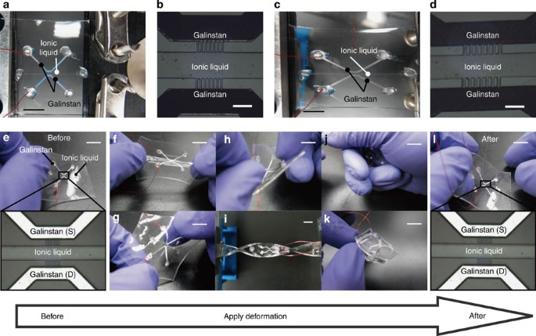Figure 3: Mechanical deformation of the liquid heterojunction device. (a,b) Optical images of a device with no strain applied using [EMIM][Otf] as the ionic liquid (a, scale bar, 5 mm;b, scale bar, 500 μm). (c,d) Optical images of the device stretched by 90% perpendicular to the axis of the junction channels, showing that the liquid confinement and heterointerface are well maintained (c, scale bar, 5 mm;d, scale bar, 500 μm). (e–l) Optical images of a device as it undergoes various forms of deformation (scale bar, 5 mm). After undergoing all the various user-applied deformations, the separation of the liquids in the channels was well maintained (l). Figure 3a–d illustrates optical images of a device undergoing 90% uniaxial strain with the liquids maintaining their confinement and junction interface. Above 90% strain, the device failed ( Supplementary Fig. 4 ), although it should be noted here that the failure was due to the solid PDMS substrate rather than that of the liquid heterojunction. Figure 3e–l demonstrates the mechanical stability of the device as it undergoes various other forms of deformation: bending ( Fig. 3h ), twisting ( Fig. 3i ), grasping ( Fig. 3j ) and tying ( Fig. 3k ). The substrate withstood all deformations and the structure of the liquid heterojunction was maintained as shown in Fig. 3l . The results demonstrate the unique feature and potential of liquid-state device technology, taking advantage of the inherent mechanical property of the liquid phase. Figure 3: Mechanical deformation of the liquid heterojunction device. ( a , b ) Optical images of a device with no strain applied using [EMIM][Otf] as the ionic liquid ( a , scale bar, 5 mm; b , scale bar, 500 μm). ( c , d ) Optical images of the device stretched by 90% perpendicular to the axis of the junction channels, showing that the liquid confinement and heterointerface are well maintained ( c , scale bar, 5 mm; d , scale bar, 500 μm). ( e – l ) Optical images of a device as it undergoes various forms of deformation (scale bar, 5 mm). After undergoing all the various user-applied deformations, the separation of the liquids in the channels was well maintained ( l ). Full size image Temperature sensing The fabricated liquid heterojunctions are electrically active and can be configured as functional devices. As a proof of concept, here we utilize our Galinstan/ionic liquid/Galinstan heterojunction device as a temperature sensor. The device operates as a temperature-sensitive constant phase element (non-ideal capacitor) and resistor in series, with the two Galinstan regions acting as the source/drain metal electrodes and the ionic liquid ([EMIM][Otf]) channel acting as the temperature-sensitive active component ( Fig. 4a ). Note that Galinstan exhibits minimal temperature response ( Supplementary Fig. 5 ) and acts as the passive element of the device. Sensing experiments were performed by placing the samples inside an oven while varying the temperature from 25 to 69 °C. Both the capacitance, C , and conductance, G , of the sensor were extracted via capacitance–voltage measurements as a function of temperature ( Supplementary Note 1 and Supplementary Fig. 6 ). 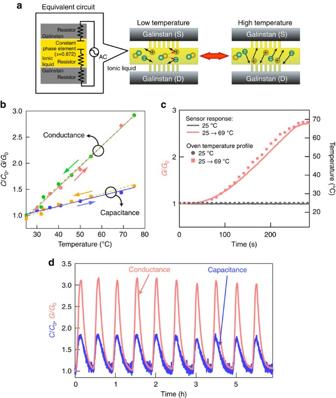Figure 4: Liquid-state heterojunctions as temperature sensors. (a) The equivalent circuit of the device. The mobility and number of dissociated ions in the ionic liquid increase with increasing temperature, which leads to an increase in conductance (middle and right schematics). (b) Measured conductance,G(red, temperature loading, green temperature unloading), and capacitance,C(blue, temperature loading, yellow temperature unloading), of the sensor as a function of temperature. The data points are normalized by the values at 25 °C (G0andC0, respectively). (c) Time-dependent measurements of the sensor (solid lines) as the oven temperature is increased (square marks). The response of the sensor closely matches the oven temperature profile, measured by a thermocouple. (d) Normalized conductance and capacitance,GandC, of the sensor for 10 temperature loading and unloading cycles (temperature cycled between 25 and 80 °C). All data are obtained using [EMIM][Otf] as the ionic liquid component of the sensors. Figure 4: Liquid-state heterojunctions as temperature sensors. ( a ) The equivalent circuit of the device. The mobility and number of dissociated ions in the ionic liquid increase with increasing temperature, which leads to an increase in conductance (middle and right schematics). ( b ) Measured conductance, G (red, temperature loading, green temperature unloading), and capacitance, C (blue, temperature loading, yellow temperature unloading), of the sensor as a function of temperature. The data points are normalized by the values at 25 °C ( G 0 and C 0 , respectively). ( c ) Time-dependent measurements of the sensor (solid lines) as the oven temperature is increased (square marks). The response of the sensor closely matches the oven temperature profile, measured by a thermocouple. ( d ) Normalized conductance and capacitance, G and C , of the sensor for 10 temperature loading and unloading cycles (temperature cycled between 25 and 80 °C). All data are obtained using [EMIM][Otf] as the ionic liquid component of the sensors. Full size image Figure 4b,c shows the temperature dependence of C and G , normalized to their values at 25 °C ( C 0 and G 0 , respectively). Both capacitance and conductance increase with temperature. Specifically, as the temperature increased from 25 to 69 °C, conductance and capacitance values increased by ~272% and 144%, respectively. Notably, the sensor response is linear for the explored temperature range of 25–69 °C with a sensitivity of 3.9% change in conductance per degree Celsius. As shown in Fig. 4b , the sensor response between temperature loading and unloading (that is, the temperature hysteresis loop) is highly identical, thus exhibiting minimal hysteresis. In addition, the response is highly stable over multiple temperature cycling ( Fig. 4d ) with a s.d. in the sensor output of <2.5% for 10 measurement cycles (temperature was cycled between 25 and 80 °C), which is within the error of the oven temperature reading. Based on the s.d. of 2.5% for multiple cycling and the sensitivity of 3.9% per degree Celsius, the minimum detectable temperature change using [EMIM][Otf] is (2.5%)/(3.9% per degree Celsius)=0.64 °C. Two other ionic liquids, [BMIM][PF6] and [BMPYR][NTf2], were also configured into a similar device structure ( Supplementary Fig. 7 ), exhibiting temperature sensitivities of 9.3% and 7.4% per degree Celsius for conductance, respectively. These results show the generic nature of our process scheme, and its compatibility with different active ionic liquids for fabrication of functional liquid-state devices. Not only can the sensitivity of a given sensor be optimized by changing the ionic liquid, but, more importantly, different chemical sensing functionality can be obtained as discussed later in this manuscript. The sensitivity of our temperature sensor compares favourably with other stretchable temperature sensors reported in literature based on solid-state materials. For instance, temperature sensors based on wrinkled [17] and wavy metal lines [6] exhibit sensitivities of ~0.2 and 0.53% per degree Celsius, respectively, for the same temperature range. In this regard, our sensor with [BMIM][PF6] as the active ionic liquid presents a 17–46 × enhancement in sensitivity over previous works. The high sensitivity of our temperature sensor is owing to the ion transport properties of the ionic liquid. The conductance of ionic liquids are known to drastically increase with temperature [27] . Ion transport is a thermally activated process [25] , with enhanced ion mobility at elevated temperatures ( Fig. 4a ). In addition, ion dissociation (that is, generation) is enhanced at high temperatures [29] , thereby leading to an increase in charge carriers ( Fig. 4a ). Both effects lead to increased conductivity with temperature. The temperature dependence of the capacitance is associated with the change in the double layer formed by the ionic liquid. The exact mechanism, however, is not well established and different explanations have been proposed in literature. One proposed explanation is that the free vacancies in the ionic liquid increase with temperature [29] . Another theoretical model has shown that complex molecules in the double layer dissociate as the temperature increases [30] . Lockett et al. [31] report that the increase in temperature causes an increase in the number of ions available for adsorption at the double layer that leads to an increase in capacitance with temperature. Nevertheless, our experimental trend of increasing capacitance with temperature is consistent with those reported in literature [29] , [30] , [31] . As can be seen in Fig. 4c , the change in conductance of our sensor quickly follows the change in temperature of the oven measured via a thermometer. This means that the measured response time of our sensor is limited by the temperature ramp time of the oven (on the order of 0.4 °C s −1 ). Deformation effects on the heterojunction sensor The stability of the sensor functionality using [EMIM][Otf] under stretching and twisting deformations is illustrated in Fig. 5 . As depicted in Fig. 5a , the conductance and capacitance increase by 13% and 8%, respectively, as the device undergoes 30% uniaxial stretch perpendicular to the axis of the junction channels. On the other hand, when the device is stretched by 30% along the axis of the junction channels, the conductance and capacitance decrease by 13% and 1%, respectively ( Supplementary Fig. 8 ). When the device is stretched perpendicular to the axis of the junction channels, the widths of the junction channels increase while their lengths decrease, leading to an increase in conductance and capacitance. However, when the device is stretched along the axis of the junction channels, the junction channels become elongated and thinner, thus leading to a drop in conductance and capacitance. The changes in conductance and capacitance of our device due to deformation are consistent with expected geometric changes in the device dimensions ( Fig. 5b and Supplementary Fig. 9 and Supplementary Note 2 ). 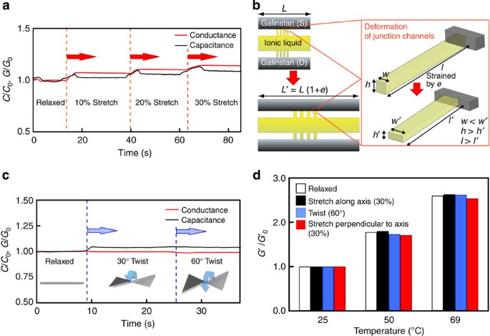Figure 5: Temperature sensing while under various modes of deformation. (a) The relative conductance and capacitance as a device is stretched by 10, 20 and 30% perpendicular to the axis of the junction channels. Here, [EMIM][Otf] is used as the ionic liquid. (b) A schematic of the relative structural change of the junction channels when the device is stretched perpendicular to the axis of the junction channels bye. eis defined to be the change in length (ΔL) divided by the original length (L) of the whole sensor. (c) The ratio of the relative conductance and capacitance of a device when twisted by 30° and 60° at 25 °C. (d) Conductance,G′of the device at 25, 50 and 69 °C as it undergoes various forms of deformation.G0′represents the conductance of the device at 25 °C for the corresponding deformation state. Figure 5c depicts the device operation when the sensor is twisted by 60° that results in a 1% drop in conductance and 4% increase in capacitance. It should be noted that the changes in C and G by strain are fully reversible. Figure 5: Temperature sensing while under various modes of deformation. ( a ) The relative conductance and capacitance as a device is stretched by 10, 20 and 30% perpendicular to the axis of the junction channels. Here, [EMIM][Otf] is used as the ionic liquid. ( b ) A schematic of the relative structural change of the junction channels when the device is stretched perpendicular to the axis of the junction channels by e. e is defined to be the change in length (Δ L ) divided by the original length ( L ) of the whole sensor. ( c ) The ratio of the relative conductance and capacitance of a device when twisted by 30° and 60° at 25 °C. ( d ) Conductance, G′ of the device at 25, 50 and 69 °C as it undergoes various forms of deformation. G 0 ′ represents the conductance of the device at 25 °C for the corresponding deformation state. Full size image We also explored the temperature sensitivity of the sensor as it is mechanically deformed. Figure 5d shows the response of conductance with respect to temperature while the device is stretched 30% along and perpendicular to the axis of the junction channels as well as twisted by 60°. Since the change caused by the deformations is significantly smaller compared with the temperature sensitivity, the sensor can operate with reasonable accuracy (up to ±2 °C error for the applied strains and temperature range) even under various forms of mechanical deformations. For practical applications, sensors can be calibrated for different deformations—matching those that they encounter for the targeted use to further enhance the sensor accuracy. For instance, standalone strain sensors based on liquid Galinstan metal lines [14] can be integrated on the same substrate. As previously reported [14] , the resistivity of patterned Galinstan lines changes with strain. Since the resistivity of Galinstan has minimal dependence on temperature, such a sensor can selectively monitor strain, thus providing a calibration pathway for the output signal of the temperature sensors as a function of strain. Humidity and oxygen gas sensing We also explored the use of liquid-state heterojunction devices for humidity and oxygen gas sensing using different ionic liquids as the active component. Previous studies have shown the high sensitivity of ionic liquids to different molecular species depending on their chemical properties. The sensitivity is often attributed to enhanced ion conductivity and/or concentration [32] , [33] . On the other hand, hydrophobic ionic liquids show minimal sensitivity to humidity, with the response decreasing with increasing hydrophobicity [34] , [35] . We observe the same trend in the conductance and capacitance of our liquid-state heterojunction devices ( Fig. 6a ). Specifically, we explored the humidity response of [EMIM][Otf], [BMIM][PF6] and [BMPYR][NTf2] with ascending hydrophobicity. [EMIM][Otf] exhibits the highest sensitivity to humidity, with a 1.7% change in conductance per 1% increase in humidity ( Fig. 6a,b ). This sensitivity is remarkably high given that the commercial humidity sensors, which are usually based on capacitive sensing, have sensitivities of ~0.3% (refs 25 , 31 ). On the other hand, [BMPYR][NTf2] shows the least response with a sensitivity of <0.2% change in conductance per 1% increase in humidity for the explored humidity range of 13–87%. This minimal sensitivity to humidity makes [BMPYR][NTf2] the more optimal ionic liquid for temperature sensing applications since the humidity level often changes with temperature. Considering the high sensitivity of [BMPYR][NTf2] to temperature as shown in Supplementary Fig. 7 , a humidity change from 13 to 87% leads to a temperature reading inaccuracy of only ±1.6 °C for this sensor. 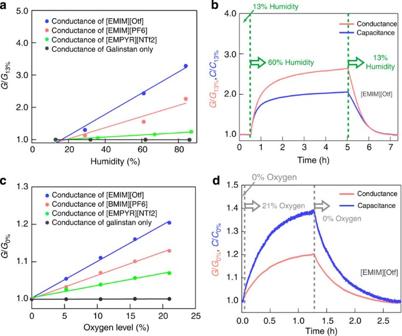Figure 6: Liquid-state heterojunctions as oxygen and humidity sensors. (a) Measured conductance of devices made with three different ionic liquids as a function of humidity. (b) Measured conductance and capacitance of a sensor with [EMIM][Otf] as the active ionic liquid for one loading and unloading cycle between 13% and 63% humidity, respectively. The data points are normalized by the values at 13% humidity and 25 °C (G13%andC13%, respectively). (c) Measured conductance of the sensor as a function of oxygen concentration. (d) Measured conductance and capacitance of a sensor with [EMIM][Otf] as the active ionic liquid for one loading and unloading loop between 0% and 21% oxygen, respectively. The data points are normalized by the values at 0% oxygen (100% nitrogen) at 25 °C (G0%andC0%, respectively). Figure 6: Liquid-state heterojunctions as oxygen and humidity sensors. ( a ) Measured conductance of devices made with three different ionic liquids as a function of humidity. ( b ) Measured conductance and capacitance of a sensor with [EMIM][Otf] as the active ionic liquid for one loading and unloading cycle between 13% and 63% humidity, respectively. The data points are normalized by the values at 13% humidity and 25 °C ( G 13% and C 13% , respectively). ( c ) Measured conductance of the sensor as a function of oxygen concentration. ( d ) Measured conductance and capacitance of a sensor with [EMIM][Otf] as the active ionic liquid for one loading and unloading loop between 0% and 21% oxygen, respectively. The data points are normalized by the values at 0% oxygen (100% nitrogen) at 25 °C ( G 0% and C 0% , respectively). Full size image Finally, the oxygen sensitivity of the liquid-state devices is examined as depicted in Fig. 6c,d . All three ionic liquids exhibit increase in conductance and capacitance in response to oxygen with [EMIM][Otf] exhibiting the highest sensitivity of 1.0% increase in conductance per 1% increase in oxygen concentration. As shown here, using different ionic liquids as the sensing element can yield tuned response to various stimuli. For each type of stimuli, the sensing can be optimized by choosing the proper ionic liquid. In the future, multiple liquid heterojunction sensors, each with a different ionic liquid may be multiplexed into a fully integrated system to sense different stimuli with calibrated response. In conclusion, the work here presents a platform for exploring liquid-state devices based on ‘heterojunctions’ of complementary liquids embedded in soft templates. Through modelling and experiments, we map the design parameters needed to enable formation of controlled liquid heterointerfaces, without intermixing. Given the inherent mechanical deformability of the liquid phase, the use of liquid-state device technology presents a natural platform for conformal electronics. Specifically, the work enables exploration of new devices that can undergo extreme levels of mechanical deformation without fracture or delamination that is often associated with solid-state materials. Moving forward, exploring the size scaling limits of the device may be of interest depending on the targeted application. Specifically, in this work, the microfluidic channels used for the injection of the liquids were 31-μm thick and 500-μm wide. However, previous reports have demonstrated fabrication of liquid channels down to ~100 nm in height and width. Thus, it should be possible to scale down the all-liquid sensors to significantly smaller dimensions than those presented in this work. Furthermore, opportunities exist in exploring a wide range of liquid heterojunctions for fabricating various sensors and electronic device components, including diodes and transistors. Overall, the work presents an important step towards the potential realization of liquid-state electronic systems that offer new form factors and functionality. Preparation of the SU-8 mould SU-8 (SU-8 2075, MicroChem) was spin-coated onto a silicon handling wafer at 500 r.p.m. for 5 s and then at 2,000 r.p.m. for 30 s ( Fig. 1a ). The SU-8 was then baked at 90 °C for 10 min and patterned using photolithography with a transparency mask. After exposure, the sample was baked again at 90 °C for 10 min followed by development using propylene glycol monomethyl ether acetate (Sigma-Aldrich). This process yielded SU-8 microchannel mould patterns ( Fig. 1b ) 31±2 μm high, measured via a three-dimensional confocal laser microscope (Olympus LEXT OLS4000). To aid in the liftoff process of the PDMS, the SU-8 mould was then treated with trichloro(1H,1H,2H,2H-perfluorooctyl)silane (Sigma-Aldrich) to prevent adhesion of PDMS to the silicon handling wafer. Temperature sensor fabrication PDMS (Sylgard 182, Dow Corning) mixed with a base to curing agent ratio of 13:1 was poured onto the SU-8 mould to a thickness of ~1 mm and cured on a hot plate at 90 °C for 10 min ( Fig. 1c ). After curing, the patterned PDMS was cut and peeled off from the SU-8 mould ( Fig. 1d ). On a separate clean glass slide, S1818 photoresist (MicroChem) was spin-coated at a speed of 4,000 r.p.m. for 30 s and then baked on a hot plate at 90 °C for 90 s. PDMS mixed with the 13:1 base to curing agent ratio was then spun onto the slide at 500 r.p.m. for 1 min yielding a PDMS thickness of ~100 μm ( Fig. 1e ). The sample was then cured on a hot plate at 50 °C for 6 h. This unpatterned substrate, along with the PDMS substrate patterned using the SU-8 mould, were both exposed to an oxygen plasma (Diener Electronic Nano) at 120 W for 90 s and then bonded together ( Fig. 1f ). Galinstan (Rotometals) was injected into the microfluidic channels using a PHD 2000 syringe pump (Harvard Apparatus) at a speed of 25–1900 μl per minute ( Fig. 1g ). The ionic liquids, [EMIM][Otf], [BMIM][PF6], [BMPYR][NTf2] or [HMIM][Cl] (Sigma-Aldrich) were then injected into the middle channel ( Fig. 1h ). To prevent bubble formation, the Galinstan and ionic liquid were injected soon after oxygen plasma treatment of the PDMS substrate so that the contact angles between the ionic liquid and PDMS were as small as possible. This allows us to obtain the highest possible capillary pressure for injection of the ionic liquid into the thin junction channels. Based on observations through a microscope, bubbles were not observed in the heterojunctions. It is expected that any small microbubbles that do form by chance will slowly diffuse out of the channels through the PDMS template, given the known permeability of PDMS to air molecules [36] . Copper wire electrodes were inserted into the openings of the channel ( Fig. 1i ) that were then sealed off with a room temperature vulcanizing silicone (RTV Sealant 734 Flowable Sealant, Dow Corning). Finally, acetone was used to remove the photoresist layer bonding the sample to the glass slide and the completed temperature sensor was peeled off ( Fig. 1j ) Analysis of the Nyquist plot The impedance of the devices were measured by a potentiostat (604C, CH Instruments). The devices were measured in a two-electrode configuration, with the reference and counter electrode leads connected together. The Nyquist plot was measured at an applied DC bias of 0 V, with a 10 mV AC voltage superimposed. The measurement frequency ranged from 1 to 100 kHz for [EMIM][Otf], and 1 to 10 kHz for [BMIM][PF6] and [BMPYR][NTf2], respectively. A model of electrolyte resistance R and double-layer capacitance C in series was used to fit the Nyquist plot. To account for the non-ideal behaviours of capacitance, a constant phase element was used instead of a capacitor. Temperature sensing measurement To measure the temperature dependence of the sensor, the fabricated device was put in an oven (Oven model 3511FS, Fisher Scientific) at room temperature, and the oven was turned on to the temperature set point after closing the oven door. The conductance and capacitance of the device were monitored using an Agilent B1500A semiconductor device analyser as the temperature ramped up to the set point. To test the effect of stretching and twisting on device performance, the temperature sensor was mounted onto a homebuilt apparatus capable of both stretching and twisting the device. The conductance and capacitance of the device was monitored as the device was stretched by up to 30% and twisted by up to 60°. When doing the temperature dependence studies of the temperature sensor while under strain, the whole apparatus containing the strained device was placed in the oven, and the conductance and capacitance were monitored as the oven temperature was increased. Oxygen sensing measurement O 2 was mixed with N 2 (99.998%) using two flowmeters to obtain the desired O 2 concentrations. The gases were flowed through a quartz tube containing the sensor with a total volumetric flow rate of 1 l min −1 . The humidity and temperature were maintained within ±1% and ±1 °C, respectively, during the measurement. Electrical measurements were performed using the same methods as for temperature sensing. Humidity sensing measurement In order to control humidity, two air lines for dry air and air with high moisture content (obtained by bubbling dry air through a water bath) were connected to a quartz tube containing the liquid-state heterojunction sensor. The total volumetric flow rate of dry and moist air was maintained at 1 l min −1 using a flowmeter. The humidity was controlled by altering the ratio of dry and moist air. The temperature and humidity were monitored by using a commercial temperature/humidity sensor (EK-H5, Sensirion). Electrical measurements were performed using the same methods as for temperature sensing. How to cite this article : Ota, H. et al. Highly deformable liquid-state heterojunction sensors. Nat. Commun. 5:5032 doi: 10.1038/ncomms6032 (2014).